The nuclear translocation of ERK1/2 as an anticancer target A hallmark of the ERK1/2 functioning is their nuclear translocation, which is mainly required for the induction of proliferation. Activated ERK1/2 molecules that remain in the cytoplasm initiate other activities, including immediate feedback loops. Prevention of the nuclear translocation should therefore inhibit proliferation, without affecting cytoplasm-induced cellular processes. Here we present an NTS-derived myristoylated phosphomimetic peptide, which blocks the interaction of importin7 and ERK1/2, and consequently the nuclear translocation of the latter. In culture, the peptide induces apoptosis of melanoma cells inhibits the viability of other cancer cells, but has no effect on non-transformed, immortalized cells. It even inhibits the viability of PLX4032- and U0126-resistant melanoma cells. In xenograft models, the peptide inhibits several cancers, and acts much better than PLX4032 in preventing melanoma recurrence. This study provides a proof of concept for using the nuclear translocation of ERK1/2 as a drug target for the combat of various ERK1/2-related cancers. The extracellular signal-regulated kinase 1/2 (ERK1/2) cascade is an intracellular signalling pathway composed of a sequential phosphorylation and activation of Raf or other MA3Ks, MEK1/2, ERK1/2 and several downstream MAPKAPKs, which regulates a large number of cellular processes including mainly proliferation and differentiation [1] , [2] , [3] . Being a central regulatory pathway, its dysregulation is involved in various pathologies and is particularly known to play a role in cancer [4] , [5] . Indeed, inhibitors of both Rafs and MEK1/2 have been recently developed for the treatment of melanoma [6] , [7] , and it is likely that specific ERK1/2 inhibitors will be developed for the same purpose as well [8] . However, despite of the widespread involvement of the ERK1/2 cascade in the induction and maintenance of cancers, the inhibitors of the cascade were proven beneficial only in B-Raf-mutated melanomas (B-Raf melanomas) [9] , [10] . In addition, most sensitive melanomas develop resistance to the Raf/MEK inhibitors within several months of treatment [11] . The lack of effect in many cancer types and the mechanisms of acquired resistance are now being investigated, and it was recently shown that in some cases these mechanisms of resistance involve the inhibition of ERK1/2-dependent negative feedback loops. Consequently, this inhibition allows hyperactivation of upstream signalling components that circumvent the inhibited ERK1/2 cascade [12] , [13] . Hence, inhibiting ERK1/2 without affecting feedback loops should result in an efficient anticancer drug. One of the key steps in the transmission of ERK1/2 signals is the nuclear translocation of ERK1/2. Indeed, in resting cells, most of ERK1/2 molecules are localized in the cytoplasm owing to their anchoring to a variety of cytosolic proteins such as cytoskeletal components and scaffold proteins [14] . Upon stimulation and activation of ERK1/2, a large portion of these proteins assumes a rapid and massive nuclear translocation [15] . The molecular mechanism of the translocation of ERK1/2 involves TEY phosphorylation-dependent conformational change, which results in detachment of the ERK1/2 molecules from their anchors [16] . This exposes ERK1/2 to an additional phosphorylation on two Ser residues within a sequence of nine amino acids termed nuclear translocation signal (NTS) located within the kinase insert domain of ERK1/2 (ref. 17 ). This phosphorylation can be mediated by both stimulated and constitutively active protein kinases, including protein kinase CKII, and autophosphorylation by active ERK1/2 themselves [18] , [19] . The phosphorylation of the NTS then allows the beta-like importin, Imp7, to bind it, and consequently induce the nuclear translocation of these kinases. This rapid and robust translocation then allows the phosphorylation and modulation of activity of a large number of nuclear proteins, which are important for the induction and regulation of cellular processes [4] , [20] . Interestingly, it was shown that the nuclear translocation of ERK1/2 is mainly important for the induction of proliferation [21] , while other ERK1/2-dependent processes are mostly regulated by the cytosolic molecules [22] . In addition, we have recently shown that the mechanism of translocation of ERK1/2 is distinct from the other mitogen-activated protein kinases (MAPKs) JNK1/2 and p38α/β (ref. 23 ). Because the nuclear translocation of ERK1/2 is mainly involved in the induction of proliferation, while many negative feedback loops are initiated by cytoplasmic ERK1/2, we hypothesized that inhibition of the nuclear translocation should inhibit proliferation without affecting cytosolic-induced processes including the induction of feedback loops. Therefore, such inhibition should be effective in many cancer types, result in less side effects and acquire less drug resistance than the currently used drugs. In this study, we used myristoylated, NTS-derived phosphomimetic peptide (EPE peptide), and found that it inhibits the interaction of importin7 with ERK1/2, and consequently the nuclear translocation of the latter. In culture, the application of the peptide induces apoptosis of melanoma cells, inhibits the proliferation/survival of many other cancer cells, and even PLX4032 and U0126-resistant melanoma cells, but has no effect on the viability of several immortalized cells. In addition, the peptide significantly reduces the phosphorylation of the ERK1/2-dependent nuclear transcription factors, Elk1, c-Myc and c-Fos, but has no significant effect on TEY-ERK1/2, SPS-ERK1/2, RSK and AKT phosphorylations. When used in xenograft models, systemic application of the peptide significantly inhibits the growth of breast cancer, colon cancer and melanoma-derived tumours, and completely eradicates the growth of low-passage melanoma tumour in severe combined immunodeficiency (SCID) mice. Moreover, the peptide is significantly more effective than PLX4032 in preventing tumour recurrence of treatment-eradicated melanoma xenografts. This study provides a proof of concept for using the nuclear translocation of ERK1/2 as a drug target for the combat of various Ras/ERK1/2-related cancers. The myr-EPE peptide inhibits nuclear translocation of ERK1/2 The nuclear translocation of ERK1/2 is a key step in mediating cellular proliferation while having only minor influence on other cellular processes. We found that the stimulated translocation of ERK1/2 requires the binding of their phosphorylated NTS with importin7. To prevent this interaction, we used an NTS-derived peptide (GQLNHILGILGSPSQED, SPS) that should compete with the binding. To be effective, the peptide should rapidly penetrate through cell membrane and remain in the cytoplasm for a certain time. To reach this goal, we examined two known ways to allow peptide penetration: modified viral TAT sequence [24] or myristic acid (Myr [25] ), both in the N terminus of the peptide. Using biotinylated peptide with either carrier, we found that both of them induce an efficient penetration into HeLa cells, while the Myr peptide remained in the cytoplasm longer than the peptide with the TAT sequence ( Supplementary Fig. 1 ). We then undertook to examine the effect of the peptide on the nuclear translocation of ERK1/2. First, we compared the efficacy of the SPS peptide to similar peptides in which the SPS motif was replaced with either phosphomimetic (EPE) or non-phosphorylatable (APA) residues. All three peptides inhibited ERK1/2 nuclear translocation, but the inhibitory effect of the EPE peptide was somewhat stronger than that of the other two ( Supplementary Fig. 2 ). This was probably due to the ability of the EPE peptide to better mimic the importin7-bound ERK1/2, and therefore, we continued our studies with this peptide only. Treatment of four transformed cells: melanoma (A2352), breast cancer (MDA-MB-231, T47D) and cervical cancer (HeLa), and two immortalized non-transformed cells: melanocytes (NHEM-Ad) and breast (HB2) with the EPE peptide prevented the stimulation-induced nuclear translocation of ERK1/2 ( Fig. 1 ). The strong effect obtained in all these cell lines points to the generality of the inhibitory effect. The same trend of inhibition was observed with subcellular fractionation as well ( Supplementary Fig. 3 ). No significant differences between the inhibition of ERK1 and ERK2 were observed ( Supplementary Fig. 4 ), and the effect was specific to ERK1/2, as the peptide affected neither the translocation of other MAPKs ( Supplementary Fig. 5 ) nor that of AKT. 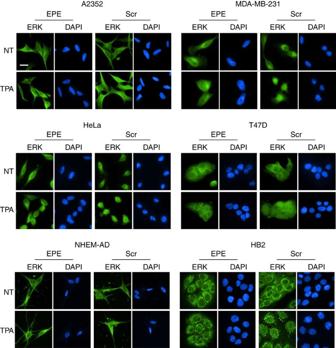Figure 1: The EPE peptide prevents nuclear translocation of ERK1/2. A2352, MDA-MB-231, HeLa, T47D, NHEM-Ad and HB2 cells were grown in full medium and then serum starved (16 h, 0.1%), pretreated either with EPE peptide, scrambled peptide (10 μM, 2 h) or DMSO control (0.1%), and then either stimulated with tetradecanoyl phorbol acetate TPA; (100 or 250 nM, 15 min) or left untreated (NT) as control. The cells were stained with αgERK1/2 Ab (c14) and DAPI. The experiments were produced three times. Scale bar, 20 μm. Figure 1: The EPE peptide prevents nuclear translocation of ERK1/2. A2352, MDA-MB-231, HeLa, T47D, NHEM-Ad and HB2 cells were grown in full medium and then serum starved (16 h, 0.1%), pretreated either with EPE peptide, scrambled peptide (10 μM, 2 h) or DMSO control (0.1%), and then either stimulated with tetradecanoyl phorbol acetate TPA; (100 or 250 nM, 15 min) or left untreated (NT) as control. The cells were stained with αgERK1/2 Ab (c14) and DAPI. The experiments were produced three times. Scale bar, 20 μm. Full size image EPE peptide effects on interactions and phosphorylations Next we undertook to identify the mechanism by which EPE peptide prevents the nuclear translocation of ERK1/2. As expected, we found that its addition to HeLa cells indeed prevented the interaction of importin7 with ERK1 when examined by co-immunoprecipitation (co-IP) with anti-importin7 antibodies (Abs) ( Fig. 2a ). We next determined the effect of the peptide on the intracellular signalling of four transformed cell lines. As expected, we detected no effect of the peptide on cytoplasmic activities including either activatory ERK1/2-TEY phosphorylation or the downstream activity of RSK ( Fig. 2b–d and Supplementary Fig. 6 ). Moreover, despite the consensus CK2-phosphorylation site the NTS phosphorylation by CK2, which occurs in the cytosol, was only moderately affected. This lack of effect supports the specificity of the peptide to ERK1/2–importin7 interaction, and may suggest that the binding sites of CK2 and importin7 to the NTS are not identical. Importantly, the peptide had no affect on the basal or stimulated phosphorylation of AKT either shortly after stimulation or in longer time periods after treatment ( Fig. 2e,f ), indicating that the negative feedback loops in the cytoplasm were not affected by the peptide. Although the peptide had no significant cytoplasmic effects, it did inhibit the phosphorylation of nuclear targets including phosphorylation ( Fig. 2b,c ) and activity ( Supplementary Fig. 7 ) of the transcription factor Elk1, the phosphorylation of c-Myc ( Fig. 2c ) and, to a lesser extent, the expression and phosphorylation of c-Fos ( Supplementary Fig. 8 ). This effect on nuclear targets varied among the cell lines (20–45% in Elk1; Fig. 2d ), and was not so pronounced for c-Fos, probably due to the involvement of other, ERK1/2-independent, signalling components in some cells. 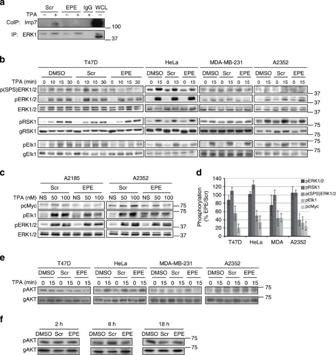Figure 2: The EPE peptide prevents interaction of ERK1 with importin7 and activation of nuclear ERK1/2 targets. (a) EPE peptide prevents ERK1/2–importin7 interaction. HeLa cells were grown in full medium and then serum starved (0.1%, 16 h), pretreated either with EPE peptide, scrambled peptide (10 μM, 2 h) or DMSO control (0.1%), and then stimulated with tetradecanoyl phorbol acetate (TPA; 250 nM, 15 min). ERK1 was precipitated from cellular extracts using αgERK1 Ab; importin7 co-IP with ERK1 was detected by western blotting with αimportin7 Ab. The closest molecular weight marker (kDa) is shown on the right of all relevant panels. (b) EPE peptide prevents Elk1, and to a lesser extent ERK1/2’s NTS, but not RSK1 phosphorylation. T47D, HeLa, MDA-MB-231 and A2352 cells were grown in full medium and then serum starved (0.1%, 16 h), pretreated either with EPE peptide, scrambled peptide (10 μM, 2 h) or DMSO control (0.1%), and then stimulated with TPA (250 nM, indicated times). Cell extracts were subjected to western blot analysis with the indicated Abs. (c) EPE peptide inhibits phosphorylation of c-Myc and Elk1 in B-Raf melanomas. A2158 and A2352 cells were grown in full medium and then serum starved (0.1%, 16 h), treated with wither scrambled or EPE peptide (10 μM, 2 h), and then stimulated with the indicated concentrations of TPA for 15 min. Cell extracts were subjected to western blot analysis with the indicated Abs. (d) Quantification of some of the results inb,c. The bars represent fold difference between scrambled and EPE peptides in the phosphorylation of the indicated proteins after TPA stimulation. The results represent the average and standard errors of two or three experiments. (e) EPE peptide does not affect short-term AKT phosphorylation. The same extracts described inbwere subjected to western blot analysis using anti-pAKT and gAKT Abs. (f) The EPE peptide does not affect long-term AKT phosphorylation. HeLa cells were treated either with EPE, scrambled peptide (10 μM) or DMSO control (0.1%) for the indicated times after which they were subjected to western blot analysis using anti-pAKT and gAKT Abs. The experiments were reproduced 2–4 times. Figure 2: The EPE peptide prevents interaction of ERK1 with importin7 and activation of nuclear ERK1/2 targets. ( a ) EPE peptide prevents ERK1/2–importin7 interaction. HeLa cells were grown in full medium and then serum starved (0.1%, 16 h), pretreated either with EPE peptide, scrambled peptide (10 μM, 2 h) or DMSO control (0.1%), and then stimulated with tetradecanoyl phorbol acetate (TPA; 250 nM, 15 min). ERK1 was precipitated from cellular extracts using αgERK1 Ab; importin7 co-IP with ERK1 was detected by western blotting with αimportin7 Ab. The closest molecular weight marker (kDa) is shown on the right of all relevant panels. ( b ) EPE peptide prevents Elk1, and to a lesser extent ERK1/2’s NTS, but not RSK1 phosphorylation. T47D, HeLa, MDA-MB-231 and A2352 cells were grown in full medium and then serum starved (0.1%, 16 h), pretreated either with EPE peptide, scrambled peptide (10 μM, 2 h) or DMSO control (0.1%), and then stimulated with TPA (250 nM, indicated times). Cell extracts were subjected to western blot analysis with the indicated Abs. ( c ) EPE peptide inhibits phosphorylation of c-Myc and Elk1 in B-Raf melanomas. A2158 and A2352 cells were grown in full medium and then serum starved (0.1%, 16 h), treated with wither scrambled or EPE peptide (10 μM, 2 h), and then stimulated with the indicated concentrations of TPA for 15 min. Cell extracts were subjected to western blot analysis with the indicated Abs. ( d ) Quantification of some of the results in b , c . The bars represent fold difference between scrambled and EPE peptides in the phosphorylation of the indicated proteins after TPA stimulation. The results represent the average and standard errors of two or three experiments. ( e ) EPE peptide does not affect short-term AKT phosphorylation. The same extracts described in b were subjected to western blot analysis using anti-pAKT and gAKT Abs. ( f ) The EPE peptide does not affect long-term AKT phosphorylation. HeLa cells were treated either with EPE, scrambled peptide (10 μM) or DMSO control (0.1%) for the indicated times after which they were subjected to western blot analysis using anti-pAKT and gAKT Abs. The experiments were reproduced 2–4 times. Full size image Effects of the peptide on cell viability Given that the nuclear activity of ERK1/2 is critical for cell proliferation, we then examined the effect of the EPE peptide on proliferation/viability of different cancer-derived and immortalized cell lines. First, we found that the optimal administration of the EPE peptide, in which it presented maximal effect on LOXIMVI and A2352 ( Supplementary Fig. 9 ), as well as HeLa and T47D cells compared with scrambled peptide control, is 10 μM every 24 h. Next, we examined the effect of the peptides on proliferation/viability of different cell lines ( Fig. 3a ). Interestingly, the response of the different cell lines to the EPE peptide can be categorized into four types. The first one was a profound reduction in cell number, which was observed in B-Raf-V600E-mutated melanoma (B-Raf melanoma). In another group, including breast, prostate and cervical cancer-derived cells, the peptide prevented additional cell growth but did not reduce it. A third group that included other melanoma, prostate and lung cancer-derived cells, presented a small decrease in cell growth as compared with a scrambled peptide control; and a fourth group that included immortalized, non-transformed cells did not respond to the peptide. Further comparison between the effects of EPE peptide and PLX4032 on the viability of some of the cell lines ( Fig. 3b ) revealed that in non-transformed melanocytes (NHEM-Ad), the EPE peptide does not have any significant effect despite the strong inhibitory effect of PLX4032. On the other hand, the EPE peptide was able to reduce the viability of the melanoma cells LOXIMVI that are not sensitive to PLX4032 as was previously reported [26] . In all other transformed cell lines examined, the effect of the EPE peptide was at least as good, or even better, than that of PLX4032. 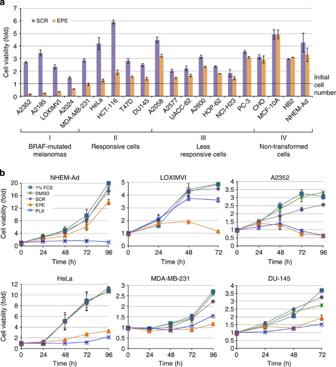Figure 3: EPE peptide prevents proliferation of cancer but not normal cells. (a) Effect of the EPE peptide on the proliferation of various cell lines. Sixteen cancer and four ‘normal’ immortalized cell lines were treated with either EPE or scrambled peptides as described above. Viable cells were quantified by methylene blue at 48 or 72 h after cell seeding. (b) Comparison of the effects of the EPE peptide and Raf inhibitor PLX4032 on cell viability. NHEM-Ad, LOXIMVI, A2352, HeLa MDA-MB-231 and DU-145 cells were treated either with EPE peptide, scrambled peptide (10 μM), PLX4032 (1 μM), DMSO control (0.1%) or no treatment at 1% fetal calf serum (FCS). Quantification of viable cells was detected as above. The graphs present the kinetic of cell growth at the indicated times. All experiments were repeated three times in triplicates. All results were presented as a fold change of the initial cell number obtained from three independent experiments and represent averages±standard errors. Figure 3: EPE peptide prevents proliferation of cancer but not normal cells. ( a ) Effect of the EPE peptide on the proliferation of various cell lines. Sixteen cancer and four ‘normal’ immortalized cell lines were treated with either EPE or scrambled peptides as described above. Viable cells were quantified by methylene blue at 48 or 72 h after cell seeding. ( b ) Comparison of the effects of the EPE peptide and Raf inhibitor PLX4032 on cell viability. NHEM-Ad, LOXIMVI, A2352, HeLa MDA-MB-231 and DU-145 cells were treated either with EPE peptide, scrambled peptide (10 μM), PLX4032 (1 μM), DMSO control (0.1%) or no treatment at 1% fetal calf serum (FCS). Quantification of viable cells was detected as above. The graphs present the kinetic of cell growth at the indicated times. All experiments were repeated three times in triplicates. All results were presented as a fold change of the initial cell number obtained from three independent experiments and represent averages±standard errors. Full size image We also compared the effect of the EPE peptide to that of the ERK inhibitor GDC-0994, which is currently in clinical trials [27] ( Supplementary Fig. 10 ). We found that the effect of the EPE peptide on cell viability was not much different than that of the ERK inhibitor in the cells examined ( Supplementary Fig. 10 ), resembling the similarity in effects to PLX4032 ( Fig. 3 ). As expected, GDC-0994 inhibited the phosphorylation of both nuclear and cytoplasmic targets, while the EPE peptide achieved its effect by partial inhibition of the nuclear target Elk1, without much change in the phosphorylation of the cytosolic target RSK ( Supplementary Fig. 10B and Fig. 2 ). Together, these results demonstrate that the EPE peptide is as good, or sometimes even better, than clinically used inhibitors of components of the ERK cascade in inhibiting proliferation of cancer cells. However, it is superior in its lack of affect on cytoplasmic negative feedback loops and on non-transformed cells. Since the intervention of the EPE peptide is downstream of the point of inhibition of B-Raf or MEK inhibitors, we next examined whether the peptide affect resistant melanoma cells. For this purpose, we generated PLX4032- and U0126-resistant cells by adding the inhibitor to A2352 melanoma cells for 6 weeks. The surviving cells proliferated slower in the presence of the inhibitors, but regained normal growth when the inhibitors were removed. Using these cells, we found that the EPE peptide was able to reduce cell viability, although this effect was not as impressive as observed in non-resistant ones ( Fig. 4a ). Similar effects were seen in two low-passage melanoma cells from vemurafenib-resistant patients ( Fig. 4b ). As expected, the EPE peptide reduced the amount of nuclear ERK1/2 both before and after stimulation ( Supplementary Fig. 11 ). No significant effects of the peptide on the activation of AKT were detected, indicating that it does not significantly affect the cytosolic negative feedback loops. Thus, our results indicate that the resistant melanoma cells are highly responsive to the EPE peptide. 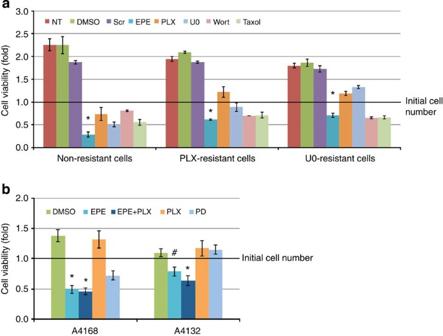Figure 4: EPE peptide prevents proliferation of MAPK inhibitor-resistant melanoma cells. (a) Melanomas that were made resistant to either PLX4032 or U0126. A2352 melanoma cells resistant to either PLX4032 or U0126 inhibitors were obtained as described under Methods section. Resistant cells were treated with the following reagents: DMSO control (0.1%), EPE or scrambled peptide (10 μM), U0126 (10 μM), PLX4032 (1 μM), Wortmannin (0.5 μM) or Taxol (25 μg ml−1), administrating fresh medium every 24 h, during the 72-h experiment. Methylene blue assay was performed to quantify viable cells. Data is presented as fold change of the initial cell number. *P<0.005 as compared with the scrambled peptide control determined by Student’st-test. (b) Resistant melanomas from patients. Two vemurafenib-resistant melanoma lines, A4132 and A4168, were grown in 1% FCS and treated with medium containing DMSO control (0.1%), EPE peptide (10 μM), PLX4032 (1 μM), PD-184352 (5 μM) or combined treatment of EPE peptide (10 μM) plus PLX4032 (1 μM), administrating fresh medium every 24 h during the 96 h experiment. Methylene blue assay was performed to quantify viable cells. *P<0.01,#P<0.05 as compared with DMSO determined by Student’st-test. All results were presented as a fold change of the initial cell number obtained from three independent experiments and represent averages±standard errors. Figure 4: EPE peptide prevents proliferation of MAPK inhibitor-resistant melanoma cells. ( a ) Melanomas that were made resistant to either PLX4032 or U0126. A2352 melanoma cells resistant to either PLX4032 or U0126 inhibitors were obtained as described under Methods section. Resistant cells were treated with the following reagents: DMSO control (0.1%), EPE or scrambled peptide (10 μM), U0126 (10 μM), PLX4032 (1 μM), Wortmannin (0.5 μM) or Taxol (25 μg ml −1 ), administrating fresh medium every 24 h, during the 72-h experiment. Methylene blue assay was performed to quantify viable cells. Data is presented as fold change of the initial cell number. * P <0.005 as compared with the scrambled peptide control determined by Student’s t -test. ( b ) Resistant melanomas from patients. Two vemurafenib-resistant melanoma lines, A4132 and A4168, were grown in 1% FCS and treated with medium containing DMSO control (0.1%), EPE peptide (10 μM), PLX4032 (1 μM), PD-184352 (5 μM) or combined treatment of EPE peptide (10 μM) plus PLX4032 (1 μM), administrating fresh medium every 24 h during the 96 h experiment. Methylene blue assay was performed to quantify viable cells. * P <0.01, # P <0.05 as compared with DMSO determined by Student’s t -test. All results were presented as a fold change of the initial cell number obtained from three independent experiments and represent averages±standard errors. Full size image The EPE peptide induces apoptosis of B-Raf melanoma cells The effect of EPE peptide on cell morphology was visualized using light microscopy. Treatment of cells with the peptide changed the appearance of B-Raf melanoma cells 24 h after treatment ( Fig. 5a ). A similar appearance, albeit a weaker one, was observed with the MEK inhibitor U0126, indicating that this effect is likely MEK1/2/ERK1/2 dependent. However, no morphological effects of the peptide were detected in most other cell types analysed ( Fig. 5a ) The change of morphology of the melanoma cells resembled cell death, which was previously reported to occur upon inhibition of the ERK1/2 cascade in B-Raf melanoma. Indeed, using TdT-mediated dUTP nick end labeling (TUNEL) ( Fig. 5b ) or PARP-1 ( Fig. 5c ) as marker for apoptosis, we found that the change in morphology correlated with an enhanced apoptosis. This apoptotic effect was specific to B-Raf melanomas, in which it was as strong as the apoptosis induced by Taxol. No apoptosis was detected in the other cell lines examined despite their clear ability to undergo a Taxol or H 2 O 2 -induced cell death. 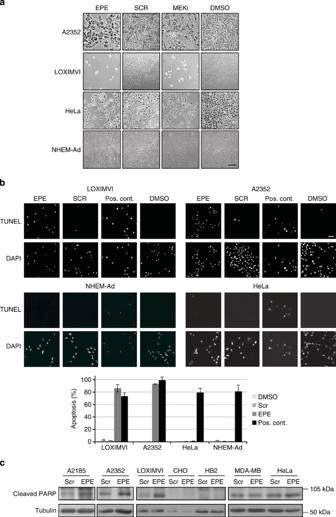Figure 5: The EPE peptide leads to apoptosis of B-Raf melanomas. (a) Effect of the EPE peptide on the morphology of A2352, LOXIMVI, HeLa and NHEM-Ad melanoma cells. The indicated cells were seeded at ~25% confluence, and treated either with EPE or scrambled peptides (10 μM), MEK inhibitors (10 μM U0126 for the first 3, and 2 μM PD-184352 for NHEM-Ad) or DMSO control (0.1%), for 48 h. Images were obtained by light microscope after 72 h. Scale bar, 50 μm. (b) Effect of the EPE peptide on the cell apoptosis determined by TUNEL staining. LOXIMVI, A2352, NHEM-Ad or HeLa cell lines were treated either with EPE or scrambled peptides (10 μM), as well as positive (pos.) control (cont.; 30 nM Taxol for LOXIMVI, A2352 and HeLa cells; 100 μM H2O2, 3 h, for NHEM-Ad) or DMSO control (0.1%) for 24 h. TUNEL staining was performed according to manufacturer’s instruction (Roche). Images were obtained and analysed by florescence microscope. Scale bar, 50 μm. The bar graph represents per cent of apoptotic cells calculated in 10 different microscopic fields. (c) Effect of the EPE peptide on cell apoptosis determined by PARP cleavage. A2352, A2185, LOXIMVI, CHO (Chinese hamster ovary), HB2, MDA-MB or HeLa cells were treated as described above, and incubated for 24 h. Cell extracts were collected and 25 μg of protein were separated by 10% SDS–PAGE. The blots were subjected to an anti-cleaved PARP Ab. The closest molecular weight marker (kDa) is shown on the right of the relevant panels. All experiments were reproduced three times. Figure 5: The EPE peptide leads to apoptosis of B-Raf melanomas. ( a ) Effect of the EPE peptide on the morphology of A2352, LOXIMVI, HeLa and NHEM-Ad melanoma cells. The indicated cells were seeded at ~25% confluence, and treated either with EPE or scrambled peptides (10 μM), MEK inhibitors (10 μM U0126 for the first 3, and 2 μM PD-184352 for NHEM-Ad) or DMSO control (0.1%), for 48 h. Images were obtained by light microscope after 72 h. Scale bar, 50 μm. ( b ) Effect of the EPE peptide on the cell apoptosis determined by TUNEL staining. LOXIMVI, A2352, NHEM-Ad or HeLa cell lines were treated either with EPE or scrambled peptides (10 μM), as well as positive (pos.) control (cont. ; 30 nM Taxol for LOXIMVI, A2352 and HeLa cells; 100 μM H 2 O 2 , 3 h, for NHEM-Ad) or DMSO control (0.1%) for 24 h. TUNEL staining was performed according to manufacturer’s instruction (Roche). Images were obtained and analysed by florescence microscope. Scale bar, 50 μm. The bar graph represents per cent of apoptotic cells calculated in 10 different microscopic fields. ( c ) Effect of the EPE peptide on cell apoptosis determined by PARP cleavage. A2352, A2185, LOXIMVI, CHO (Chinese hamster ovary), HB2, MDA-MB or HeLa cells were treated as described above, and incubated for 24 h. Cell extracts were collected and 25 μg of protein were separated by 10% SDS–PAGE. The blots were subjected to an anti-cleaved PARP Ab. The closest molecular weight marker (kDa) is shown on the right of the relevant panels. All experiments were reproduced three times. Full size image The peptide prevents the growth of human tumour xenografts We then examined the effect of the EPE peptide on the growth of tumours in xenograft models ( Fig. 6 ). For this purpose, we allowed the xenografts to grow to a size of ~60 mm 3 , and only then systemically administrated the peptide by injecting it to the tail vein of the mice. Using such xenograft models in nude mice, we found a dose-dependent inhibition of the growth of MDA-MB-231, LOXIMVI and to some extent also on HCT-116. Remarkably, an even stronger effect of the peptide was seen with a xenograft of the low-passage A2352 B-Raf melanoma in SCID mice. In this model, the peptide completely eradicated the melanoma tumour within 2 weeks of tail-vein administration. None of the animals treated exhibited any significant change in weight or other toxicity-related effects. Moreover, the treatment did not affect the size or structure of the kidneys, livers or hearts that were inspected at the end of the experiment. Interestingly, the structure of the lungs was not affected as well, although we did observe metastatic foci in lungs of vehicle- and scrambled peptide-treated, but not in EPE peptide-treated mice. 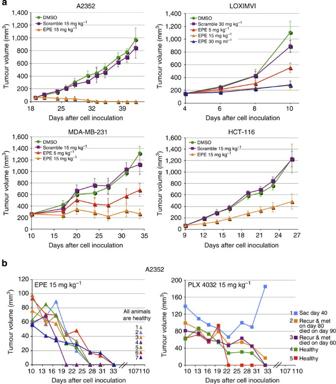Figure 6: The EPE peptide prevents the growth and tumour recurrence of human tumour xenograph in immunocompromised mice. (a) Effect of the EPE peptide on growth of four different xenograft models. CD-1 nude mice were inoculated subcutaneously with tumorigenic dose of MDA-MB-231, LOXIMVI and HCT-116 cells, and SCID mice were inoculated with A2352 cells. Upon the establishment of tumours, the mice were treated intravenously with either the EPE or scrambled peptides in the indicated doses, three times a week. Control group received an initial volume of DMSO. Tumours size was measured with a caliper and the volumes were calculated accordingly. Results were presented as averages±standard errors.n=5 per group. (b) The EPE peptide prevents tumour recurrence on melanoma xenografts. SCID mice were inoculated with A2352 cells. Upon establishment of tumours, mice were treated intravenously with EPE peptide (n=7) or intraperitoneally with PLX4032 (n=5), at the indicated doses, three times a week. Tumour size was recorded at the same time using a caliper. Following 3 weeks of treatment, mice were kept for further evaluation, monitoring for any tumour recurrence of the EPE-responsive melanoma xenografts. Experiment was concluded 110 days post inoculation (11 weeks after the last treatment) and the overall state of the animals was evaluated. Sac, sacrificed, recur, recurrence, met, metastasis. All experiments were reproduced 1–3 times. Figure 6: The EPE peptide prevents the growth and tumour recurrence of human tumour xenograph in immunocompromised mice. ( a ) Effect of the EPE peptide on growth of four different xenograft models. CD-1 nude mice were inoculated subcutaneously with tumorigenic dose of MDA-MB-231, LOXIMVI and HCT-116 cells, and SCID mice were inoculated with A2352 cells. Upon the establishment of tumours, the mice were treated intravenously with either the EPE or scrambled peptides in the indicated doses, three times a week. Control group received an initial volume of DMSO. Tumours size was measured with a caliper and the volumes were calculated accordingly. Results were presented as averages±standard errors. n =5 per group. ( b ) The EPE peptide prevents tumour recurrence on melanoma xenografts. SCID mice were inoculated with A2352 cells. Upon establishment of tumours, mice were treated intravenously with EPE peptide ( n =7) or intraperitoneally with PLX4032 ( n =5), at the indicated doses, three times a week. Tumour size was recorded at the same time using a caliper. Following 3 weeks of treatment, mice were kept for further evaluation, monitoring for any tumour recurrence of the EPE-responsive melanoma xenografts. Experiment was concluded 110 days post inoculation (11 weeks after the last treatment) and the overall state of the animals was evaluated. Sac, sacrificed, recur, recurrence, met, metastasis. All experiments were reproduced 1–3 times. Full size image In order to verify that the EPE peptide indeed operated by preventing the nuclear translocation, we stained sections of xenograft tumours, excised from the treated animals at the end of the experiments, with anti-ERK1/2 Ab. As expected, we found that EPE peptide did prevent such translocation in the treated MDA-MB-231 and LOXIMVI xenografts. In samples from the control-treated xenografts, we found ERK1/2 all over the cells with some preference to the nucleus, while in the EPE peptide-treated xenografts, ERK1/2 was localized almost exclusively in the cytoplasm ( Supplementary Fig. 12 ). These findings support the notion that the cytoplasmic retention of ERK1/2 is the cause for the specific effect of the EPE peptide. Therefore, the prevention of the nuclear translocation of ERK1/2, which does not affect the cytoplasmic activity of the cascade, may serve as an efficient tool to prevent cancer growth, with less side effects than the currently used inhibitors of the ERK1/2 cascade. The major problem with the use of B-Raf and MEK inhibitors in the clinic is the development of resistance after 6–8 months, which results in tumour and metastasis recurrence [11] . In order to study the recurrence of the disease after EPE peptide in comparison with PLX4032 treatment, we treated mice bearing A2352 xenografts with both reagents. Both treatments were proven beneficial in reducing the size of the initial ~80 mm 3 tumours. Treatment of the EPE peptide resulted in a complete disappearance of the tumours of all mice within 10–23 days ( Fig. 6b ), while the PLX4032 treatment resulted in a complete disappearance in three mice (13–23 days after treatment), and two mice with small tumours. Following last treatment administration, mice were kept for further follow-up and evaluation of melanoma condition for up to 11 weeks. None of the EPE peptide-treated mice ( N =7) showed any tumour recurrence, and all of them, as well as five other animals in a repeating experiment, remained healthy up to 11 weeks after treatment. On the other hand, as expected, in some (three out of five) of the PLX4032-treated mice the tumour did recur, and one of them appeared to develop resistance within 13 days of treatment and exhibited a massive tumour growth thereafter. These results indicate that the EPE peptide treatment may prevent resistance and tumour recurrence better than PLX4032. It is well known that ERK1/2 signalling plays a crucial role in the induction of proliferation, as well as cancer development and progression [4] . Therefore, it is not surprising that inhibitors of the ERK1/2 cascade (for example, vemurafenib and trametinib [6] , [7] ) serve as anticancer drugs. However, the majority of these agents have only a limited effect on human malignancies, and even the most effective inhibitors influence only a limited number of cancers [28] . In addition, these inhibitors may have serious side effects such as the induction of skin cancer [9] , and the treated cancers (that is, melanoma) develop resistance to the drugs within 6–8 months [11] . However, the centrality of the ERK1/2 cascade suggests that drugs that may overcome the problematic issues of the currently used inhibitors should be beneficial. Much of the shortcomings of the current inhibitors are probably mediated by reduced negative feedback loops. Therefore, we sought to prevent ERK1/2-dependent proliferation, without affecting cytosolic negative feedback loops induced by it, through the inhibition of its nuclear translocation. Indeed, the NTS-derived, EPE peptide efficiently and specifically inhibited the interaction of ERK1/2 with importin7, and thereby the nuclear translocation of ERK1/2, without changing AKT activity, which is enhanced by inhibition of the cytosolic ERK1/2-related negative feedback loops. Therefore, we undertook to analyse the peptide as a proof of concept for use of the nuclear translocation of ERK1/2 as a new target for anticancer therapy. Interestingly, although the peptide did inhibit the stimulated nuclear translocation of ERK1/2 in all cell lines examined, including non-transformed cells, its effect on cell proliferation varied. The most notable effect of the peptide was on B-Raf melanoma cells, which underwent apoptosis a few hours after treatment. This effect is similar to the apoptosis detected in B-Raf melanomas treated with B-Raf inhibitors, in which it is mediated mainly by the suppression of Bim [29] , but also involve suppression of Bmf expression and activity [30] , as well as induction of endoplasmic reticulum (ER) stress [31] . It is likely that the EPE peptide operates in a similar manner, mainly by inhibiting the ERK1/2-dependent induction of Bim and Bmf expression, which occurs in the nucleus. In addition, and probably to a lesser extent, the EPE peptide might also induce apoptosis through the induction of ER stress that is a cytoplasmic process. It should be noted that, as reported for the ERK1/2 cascade inhibitors, the apoptosis induced by the EPE peptide was specific to B-Raf melanoma, and was not observed in other melanoma types or in other cancers with mutated B-Raf ( Fig. 3 ). The reason of the lack of apoptosis in the other cells is probably owing to the fact that they are not as addicted to the ERK1/2 cascade as much as the B-Raf melanoma [32] . However, the mechanism that allows this effect specifically in the latter cells is still not clear. In addition to the pronounced effect of the EPE peptide on cell viability of melanoma cells, it had variable inhibitory effects on the growth of additional cell types. Thus, the peptide blocked the growth of several lines including MDA-MB-231, T47D and HeLa, arresting them in G1 phase of the cell cycle. On the other hand, the growth inhibition of other cell types was not as impressive and in some of them amounted only to 20–30%. The reason for this variability is not clear, as we could not find any common denominator between the cell lines in each group. It is possible though that some of the difference stemmed from an increased clearance of the peptide from the cells by the multidrug resistance (MDR) system, or from faster degradation of the peptide by proteinases. Finally, we found that the non-transformed cells examined were not sensitive to the peptide at all. This is an encouraging result that may suggest that the EPE peptide may have a good therapeutic window by affecting only the cancer but not the surrounding cells. The molecular mechanism that causes this resistance of non-transformed cells is likely dependent on the smaller number of nuclear pores and importins, which results in a slower kinetic of nuclear translocation [33] , and thereby probably a lower susceptibility to inhibition of translocation. One of the main mechanisms that mediate the resistance of cells to inhibitors of ERK1/2 signalling cascades is the lack of the ERK1/2-dependent feedback loops that render hyperactivation of other signalling components [34] , [35] . A major pathway affected by the lack of feedback loops is the PI3K-AKT, which is hyperactivated upon reduction in ERK1/2 activity in various cells [36] . The mechanisms that are involved in this activation are not fully elucidated yet, but may involve several layers of cytoplasmic regulation [37] including the inhibition of PTEN [38] . Since the negative feedback loops and the cross-talk with the AKT pathway are mainly mediated by the cytoplasmic ERK1/2 activity, we predicted that the prevention of nuclear ERK1/2 translocation would not affect it. Indeed, we found that the EPE peptide does not affect much the phosphorylation of AKT, which is indicative to the lack of effect on the ERK1/2-dependent negative feedbacks loops, in any of the cells examined. This was true not only for the short-term activation but also in later time points. The fact that AKT activity was not affected, suggesting that the EPE peptide might affect a larger number of cell lines than the Raf and MEK inhibitors. However, our results indicate that, similarly to the other inhibitors, the EPE peptide is most effective primarily in melanoma, probably because of the induction of apoptosis, which is a unique feature of ERK1/2 inhibition in this cancer. Despite this similarity, the EPE peptide has a number of advantages over the clinically approved PLX4032. First, the EPE peptide does not affect the viability of all non-transformed cells examined, including melanocytes, while PLX4032 did inhibit their growth ( Fig. 3 ). Second, the spectrum of action of the EPE peptide is wider than that of PLX4032 (for example, LOXIMVI and MDA-MB-231; Fig. 3b ). Third, the effect of the EPE peptide on xenografts of B-Raf melanoma was faster than that of PLX4032 ( Fig. 6b ). Fourth, there was no recurrence of B-Raf melanoma in the EPE peptide-treated mice, while most of the PLX4032-treated mice exhibited such a recurrence. Finally, the EPE peptide inhibited the viability of PLX4032-resistant melanomas. Thus, the use of inhibitors of ERK1/2 nuclear translocation might have an advantage over the clinically approved drugs as a first line of treatment in various cancers, and may be used as a second line therapy for vemurafenib/trametinib refractory patients. In summary, we show here that the nuclear translocation of ERK1/2 can be inhibited in most cell types using NTS-derived peptides. The peptide containing phosphomimetic residues in the NTS (EPE) was shown to have the best activity on the nuclear translocation. When administrated to cells, the EPE peptide caused apoptosis in B-Raf melanoma cells, while it had a varying grade of effect on other cancer cell types, but not on immortalized cells. The EPE peptide had no detectable effect on the ERK1/2-derived feedback loops, indicating that the effect of ERK1/2 inhibition in melanoma is mainly due to the induction of apoptosis, while in other cells this inhibition causes G1 arrest that can be overcome not only by the lack of feedback loops but also by other mechanisms. Importantly, the peptide was also shown to be very effective in xenograft models, and no recurrence of melanoma was detected in any of the animals examined. This provides a proof of concept for our assumption that the inhibition of ERK1/2 translocation to the nucleus may serve as an important tool in combatting melanoma and possibly other types of cancer. The specificity of the peptide towards the nuclear activity of ERK1/2, and the lack of effect on the immortalized cells indicate that the peptide will have much less side effects than the currently used ERK1/2-related drugs. Reagents and Abs Tetradecanoyl phorbol acetate (TPA), epidermal growth factor (EGF), Avidin-FITC (fluorescein isothiocyanate) and 4',6-diamidino-2-phenylindole (DAPI), 3,3′-diaminobenzidine (DAB) were obtained from Sigma (St Louis, MI). Anti-general Elk1 (I-20; gElk1, dilution 1:1,000), phosphorylated Elk1 (B-4, S383; pElk-1, 1:1,000), gRSK1 (C-21; 1:4,000), pRSK1/2 (T359, S381; 1:2,000), p-c-Myc (T58, S62; 1:1,000) and tubulin (1:5,000) Abs were obtained from Santa Cruz Biotechnology (CA, USA). Anti-PARP-1 (1:1,000) and pAKT (S473; 1:5,000) Abs were obtained from Cell Signaling Technology (Beverly, MA, USA). Anti-importin7 (1:3,000) Ab was obtained from Abnova (Taipei, Taiwan). Anti-pERK1/2 (pTEY-ERK), gERK1/2, gAKT1, gp38, pp38 (TGY), gJNK and pJNK (TPY) Abs were obtained from Sigma (Rehovot, Israel). Anti-gcFos (1:10,000) and anti-pcFos (T325) (1:2,000) were obtained from Abcam (Cambridge, UK). Anti-phospho SPS-ERK1/2 (1:500) Abs were produced in Biological Service Unit of the Weizmann Institute of Science (Rehovot, Israel). Secondary fluorescent Ab conjugates were obtained from Jackson ImmunoResearch (West Grove, PA). Secondary Ab conjugated to peroxidase (Simple Stained Max) was obtained from Nichirei Biosciences (Japan). Peptides The four peptides used were: (i) Scramble—GNILSQELPHSGDLQIG, (ii) SPS—GQLNHILGILGSPSQED, (iii) APA—GQLNHILGILGAPAQED and (iv) EPE -GQLNHILGILGEPEQED. Each of them was conjugated in its N-terminal to either a modified TAT sequence (YARAAARQARA; ref. 24 ), or myristic acid [25] and C-terminal amidated. To study the rate of absorption, the two SPS peptides were conjugated to lysine–biotin in their C terminus. All peptides were purchased from either Peptide 2 (Chantilly, VA, USA) or Gnenscript (Piscataway, NJ, USA). The peptides were >85% pure and kept as 100 mM dimethylsulphoxide (DMSO) stock solution at −20 °C. Cells HeLa (derived from cervical cancer), MDA-MB-231 (Ras-transformed breast cancer), T47D (Her2- and Ras-negative breast cancer), DU-145 (prostate cancer), PC-3 (prostate cancer) cells were grown in either Dulbecco’s modified Eagle’s medium (DMEM) or Roswell Park Memorial Institute medium (RPMI). Immortalized, non-transformed, Chinese hamster ovary cells were grown in DMEM/F12. All of the above media were supplemented with 10% fetal calf serum (FCS). All these cell lines were obtained from ATCC (Manassas, Virginia USA). HCT-116 (colon cancer), UACC-62 (stable melanoma line with B-Raf and many other oncogenic mutations), HOP62 (lung cancer) and NCI-H23 (lung cancer) cells were obtained from NCI-60 purchased by the Biological Service Unit of our Institute. NHEM-Ad cells (normal human melanocytes; Clonetics/Lonza, MD, USA) were grown in melanocyte basal medium-4 supplemented accordingly to MGM-4 bulletkit (Lonza). Low-passage (<10) primary melanoma cells with B-Raf mutation (A2185, A2352, A2024, A2577 and A2600), low-passage vemurafenib-resistant melanoma cells from patient (A4132 and A4168), as well as immortalized, non-transformed breast cells (HB2) were from the Ella Institute, Sheba Medical Center, Israel. Established melanoma cell line carrying B-Raf mutation, LOXIMVI, was from ATCC, and A2058 cells were kindly provided by Professor Sabatini, (MIT, Boston). These melanoma cells were grown in RPMI with 10% FCS. HB2 cells were grown in the same medium with 10 μg ml −1 insulin and 0.5 μg ml −1 hydrocortisone. A4132 and A4168 cells were grown in RPMI 15% FCS supplemented with 25 mM HEPES and 1 mM Na-pyruvate. Immortalized, breast MCF-10A cells (ATCC) were grown in DMEM/F12, 5% horse serum, 20 ng ml −1 epidermal growth factor, 10 μg ml −1 insulin, 0.5 μg ml −1 hydrocortisone and 100 ng ml −1 cholera toxin (Sigma, Israel). Fluorescence microscopy Cells were fixed in 3% paraformaldehyde in PBS for 15 min, and then permeabilized and blocked with 0.1% Triton X-100 in 2% BSA/PBS for 15 min at 23 °C. The fixed cells were sequentially incubated with appropriated Abs, (1:100 in 2% BSA/PBS, 1 h), followed by either Cy-2 or rhodamine-conjugated secondary Abs and DAPI (1:100 in 2% BSA/PBS, 1 h). To follow the subcellular localization of the biotin-conjugated peptides, cells were incubated with Avidin-FITC (1:400 in 2% BSA/PBS) and DAPI. Slides were analysed and photographed by a fluorescence microscope (Nikon, Japan, × 600). Western blotting and co-immunoprecepitation (i) Preparation of cellular extracts for western blotting: Cells were rinsed twice with ice-cold FCS and scraped into radio-immunoprecipitation assay (RIPA) buffer (137 mM NaCl, 20 mM Tris (pH 7.4), 10% glycerol, 1% Triton X-100, 0.5% deoxycholate, 0.1% SDS, 2 mM EDTA, 1 mM phenylmethylsulfonyl flouride (PMSF) and 20 μM leupeptin). The extracts were centrifuged (20,000 g , 15 min, 4 °C), and the supernatants were further analysed by western blotting. The blots were developed with horseradish peroxidase-conjugated anti-mouse or anti-rabbit Abs. (ii) Co-IP: Cells were rinsed twice with ice-cold PBS and scraped into buffer H (50 mM β-glycerophosphate (pH 7.3), 1.5 mM EGTA, 1 mM EDTA, 1 mM dithiothreitol, 0.1 mM sodium vanadate, 1 mM benzamidine, 10 μg ml −1 aprotinin, 10 μg ml −1 leupeptin and 2 μg ml −1 pepstatin). The extracts were sonicated (50 W, 2 × 7 s) and centrifuged (20,000 g , 15 min, 4 °C). Cellular extracts were incubated (2 h, 4 °C) with the appropriate Abs preconjugated to A/G beads (1 h, 23 °C). Subsequently, the beads were washed three times with co-IP washing buffer (20 mM HEPES, pH 7.4, 2 mM MgCl 2 , 2 mM EGTA, 150 mM NaCl and 0.1% Triton) and once with PBS, and subjected to western blot analysis. Morphology and apoptosis (TUNEL) assays Cells were seeded on glass cover slips in a 12-well plate at 25% confluence with medium containing 1% of FCS. Peptides (EPE or scrambled), DMSO or U0126 in a final concentration of 10 μM were added after 4 h (considered as time ‘0’). TUNEL staining was performed at 24 h after the treatment according to manufacturer’s instruction (Roche Applied Science, Nutley, NJ, USA). Briefly, the medium was removed and cells were fixed with 3% of paraformaldehyde for 1.5 h at 23 °C. Cells were rinsed twice with PBS and permeabilized with 0.1% Triton X-100 and 0.1% sodium citrate for 2 min on ice. Cells were rinsed twice with PBS and 28 μl of TUNEL reaction mixture (25 μl of TUNEL label, 2.5 μl of TUNEL enzyme and 0.1 mg ml −1 of DAPI) was added directly on top of the slide, cells were incubated for overnight in a humid box at 37 °C. Cover slips were rinsed three times with PBS and mounted on microscope slides. The slides were dried and then subjected to image acquisition by a fluorescence microscope. For morphology assay, the cells were seeded at ~25% confluence in 6 cm plates with medium containing 1% FCS. EPE and scrambled peptides, DMSO or U0126 in a final concentration of 10 μM, were added after 4 (considered as time ‘0’), 24 and 48 h. Images were obtained using a light microscope (Olympus BX51) after 72 h. Viability assay All cells, except of MCF-10A, were seeded into 12-well cell plates in 1% FCS medium. MCF-10A cells were seeded in their complete medium diluted fivefold. DMSO, scrambled peptide, EPE peptide, U0126 (final concentration of 10 μM each) or PLX4032 (1 μM) were added to the appropriated wells 4 h later. Fresh medium containing the same agents was replaced every day. The number of viable cells was measured by methylene blue assay at 72 or 96 h after cell seeding. Shortly, cells were fixed with 4% formaldehyde for 2 h at 23 °C, washed once with 0.1 M borate buffer pH 8.5 and stained with of 1% methylene blue in 0.1 M borate buffer for 10 min. Colour was extracted by adding 0.1 M HCl (3 h, 23 °C) and was examined at 595 nm. For time course experiments, viable cells were measured at 0, 24, 48, 72 and 96 h after cell seeding. For dose–response experiments, we treaded cells with 0.1, 1, 3, 10 or 30 μM of peptides for 72 h as above. Studies on inhibitors-resistant melanoma cells A2352 cells were supplemented with either PLX4032 (B-Raf inhibitor, 1 μM), or U0126 (MEK inhibitor, 10 μM) for 45 days. Cells that survived this inhibitory pressure were treated with the following agents: DMSO, scrambled peptide, EPE peptide, U0126 (final concentration of 10 μM each), PLX4032 (1 μM), Wortmannin (PI3K inhibitor, 0.5 μM) or Taxol (25 ng ml −1 ), and subjected to proliferation assay as described above. Animal studies All animal experiments were approved by the Animal Care and Use Committee of the Weizmann Institute of Science (Rehovot, Israel). Female CD-1 nude mice (Harlan), 5–6 weeks of age, were inoculated subcutaneously into the flank region with 2 × 10 6 MDA-MB-231, LOXIMVI, or HCT-116 cells in 150 μl PBS. Female SCID mice (Harlan), 5–6 weeks of age, were inoculated subcutaneously into the flank region with 10 7 A2352 cells in 150 μl mixture of PBS with Matrigel (2:1). Tumours were allowed to develop to the size of 5–6.5 mm in diameter (50–110 mm 3 volume) and then the animals were randomly allocated to different treatment groups. The peptides (100 mM stock in DMSO) were diluted to the necessary concentration in PBS and boiled for 5 min. DMSO, scrambled or EPE peptides were administered by intravenous injection into the tail vein (150 μl per mouse, three times a week). PLX4032 was dissolved in 2% methylcellulose and injected intraperitoneally (three times a week). Tumour dimensions were measured with a caliper. Tumour volume was calculated using: V = D 1 × D 2 × D 3 × π /6, where D 1 , D 2 and D 3 represent the three mutually orthogonal growth diameters. To assess any signs of systemic toxicity, body weight was monitored and recorded at the end of the experiment. Histology and immunohistochemistry Tumour xenografts, lungs, livers, kidney and hearts of animals from different treatment groups were removed and subjected to histological analysis by staining of 5 μm paraffin-embedded tissue slides with haematoxylin and eosin, and examination by light microscope. MDA-MB-231 and LOXIMVI tumour xenografts were subjected to immunohistochemical analysis using αgERK Abs. Briefly, paraffin-embedded blocks of tumours after different treatments were cut at 4 μm thickness and stained with ERK1/2 Abs, followed by secondary Abs conjugated to peroxidase and 3,3′-diaminobenzidine staining. Representative fields of each specimen were photographed at × 20 and × 40 magnifications. How to cite this article: Plotnikov, A. et al . The nuclear translocation of ERK1/2 as an anticancer target. Nat. Commun. 6:6685 doi: 10.1038/ncomms7685 (2015).